Plasmonic nanoresonators for high-resolution colour filtering and spectral imaging Colour and spectral imaging systems typically use filters and glass prisms to disperse light of different wavelengths. With the miniaturization of integrated devices, current research on imaging sensors focuses on novel designs aiming at high efficiency, low power consumption and slim dimension, which poses great challenges to the traditional colourant-based filtering and prism-based spectral splitting techniques. In this context, surface plasmon-based nanostructures are attractive due to their small dimensions and the ability to efficiently manipulate light. In this article we use selective conversion between free-space waves and spatially confined modes in plasmonic nanoresonators formed by subwavelength metal–insulator–metal stack arrays to show that the transmission spectra through such arrays can be well controlled by using simple design rules, and high-efficiency colour filters capable of transmitting arbitrary colours can be achieved. These artificial nanostructures provide an approach for high spatial resolution colour filtering and spectral imaging with extremely compact device architectures. In recent years, surface plasmons (SPs) and related plasmonic nanostructures have generated considerable interest with the development of nanofabrication and characterization techniques [1] , [2] , [3] , [4] , [5] , [6] , [7] . SPs are essentially charge density waves generated by the coupling of light to the collective oscillation of electrons on the metal surface [8] . By exploiting plasmonic nanostructures, such as nanohole or nanoslit arrays, efficient conversion between photons and plasmons can be controlled at subwavelength scale, which may provide new solutions to traditional optical processes such as colour filtering and spectral imaging [9] , [10] . Recently, such effects have been reported using a metallic nanohole array to filter colour by tuning the resonant transmission peak at the visible range [5] , [11] . However, the transmission passbands of such filters are relatively broad and do not satisfy the requirement for the multiband spectral imaging. Other attempts such as nanoslits combined with period grooves [12] or inserted into a metal–insulator–metal (MIM) waveguide [13] also show colour filtering effect. However, in these structures, two neighbouring output slits must be separated by additional structures or by specific coupling distances (both about several micrometres, causing attenuation due to metal absorption loss); therefore, the device dimension and efficiency are restricted. Moreover, because of the thick metal film used in these structures, the absorption loss from light entering and leaving the MIM waveguide further decreases the devices' efficiencies to generally <10%. Such a value does not satisfy the requirement for practical display applications. Among these efforts, the filters generated by MIM waveguide resonators are of particular interest. MIM waveguide geometries offer the ability to support SP modes at visible wavelengths and have been widely investigated for different applications, such as guiding waves at subwavelength scale [14] , [15] , [16] , [17] , concentrating light to enhance the absorption for photovoltaic applications [18] , [19] , [20] , providing a near-field plate for superfocusing at optical frequency [21] or composing metamaterials for strong magnetic resonance and negative refraction [22] , [23] , [24] , [25] . Besides enabling efficient subwavelength confinement of spatial modes, compared with other nanostructures, the top and bottom metal layers of MIM waveguides can be integrated as electrodes in a straightforward manner in the electro-optic system, both of which can compact the device size. We report herein the design and demonstration of plasmonic MIM nanoresonator structures capable of filtering white light into individual colours across the entire visible band. The design principle can also be applied to other wavelength ranges. The key concept here is to use nanoresonators to realize the photon–plasmon–photon conversion efficiently at specific resonance wavelengths. Compared with the aforementioned colour-filtering methods, our new design significantly improves absolute transmission, pass bandwidth and compactness. In addition, the filtered light is naturally polarized, making it very attractive for direct integration in liquid crystal displays (LCDs) without a separate polarizer layer [26] . 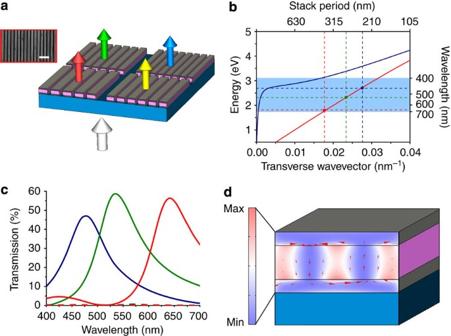Figure 1: Plasmonic nanoresonators formed by MIM stack arrays. (a) Schematic diagram of the proposed plasmonic nanoresonators. The white arrow represents the incident white light and the red, yellow, green and blue arrows represent the transmitted coloured light from the different stack arrays. Grey, pink and blue in the structure indicate the material of aluminium, zinc selenide and magnesium fluoride respectively. Inset is the scanning electron microscopy image of the fabricated device. Scale bar, 1 μm. (b) Plasmon dispersions in MIM stack array. Red, green and blue dots correspond to the case of filtering primary RGB colours. Red and blue curves correspond to antisymmetric and symmetric modes respectively. The shaded region indicates the visible range. (c) Simulated transmission spectra for the RGB filters. The solid and dash curves correspond to TM and TE illuminations respectively. The stack period for RGB filters is 360, 270 and 230 nm. (d) Cross-section of the time-average magnetic field intensity and electric displacement distribution (red arrow) inside the MIM stack at a wavelength of 650 nm with 360 nm stack period. The colours on the right side represent the constitutive materials, defined as ina. Plasmonic nanoresonators for colour filtering Figure 1a presents the schematic diagrams of the proposed nanoresonators. For easy fabrication, the device is designed as a subwavelength periodic MIM stack array on a magnesium fluoride (MgF 2 ) transparent film with period P . For each stack, a 100 nm-thick zinc selenide (ZnSe) layer is sandwiched by two 40 nm-thick aluminium (Al) layers, wherein the thickness of the dielectric core is determined on the basis of the spatial extension of SP waves inside the ZnSe layer at the visible frequencies [8] . The 100 nm-thick ZnSe layer ensures the efficient coupling of SP modes at the top and bottom edges of the stack, whereas the 40 nm-thick Al layer prohibits the direct transmission of the incident light. The duty cycle of the stack array is about 0.7. The bottom Al grating is used to couple selectively the incident light into plasmon waveguide modes by diffraction, whereas the top Al grating efficiently reconverts the confined plasmons to propagating waves by scattering and transmits the light to the far field in the forward direction. Figure 1: Plasmonic nanoresonators formed by MIM stack arrays. ( a ) Schematic diagram of the proposed plasmonic nanoresonators. The white arrow represents the incident white light and the red, yellow, green and blue arrows represent the transmitted coloured light from the different stack arrays. Grey, pink and blue in the structure indicate the material of aluminium, zinc selenide and magnesium fluoride respectively. Inset is the scanning electron microscopy image of the fabricated device. Scale bar, 1 μm. ( b ) Plasmon dispersions in MIM stack array. Red, green and blue dots correspond to the case of filtering primary RGB colours. Red and blue curves correspond to antisymmetric and symmetric modes respectively. The shaded region indicates the visible range. ( c ) Simulated transmission spectra for the RGB filters. The solid and dash curves correspond to TM and TE illuminations respectively. The stack period for RGB filters is 360, 270 and 230 nm. ( d ) Cross-section of the time-average magnetic field intensity and electric displacement distribution (red arrow) inside the MIM stack at a wavelength of 650 nm with 360 nm stack period. The colours on the right side represent the constitutive materials, defined as in a . Full size image For TM-polarized waves (the E -field is perpendicular to the Al grating direction), the transverse magnetic plasmon dispersion of the Al/ZnSe/Al stack array is plotted in Figure 1b . Here we only consider the normal incidence and therefore the stack period is related to the plasmon transverse wavevector as P =2 π / k x by the ±1 st order diffraction. From this figure, it can be clearly seen that the SP antisymmetric mode has a near-linear dispersion across the whole visible range. Therefore, the SP antisymmetric modes can be used as intermediates to couple the incident plane wave selectively in and scatter the confined SP modes out to the far field. The close-to-linear dispersion made it very easy to design filters for any colours across the entire visible band. As an example, the red, green and blue spots in Figure 1b represent the three primary RGB colours. They have different transverse wavevectors that correspond to specific stack periods by the ±1 st order diffraction. The simulated transmission spectra for RGB colours are shown in Figure 1c . The corresponding period of the stack is 360, 270 and 230 nm, which is well within the reach of current micro- and nanofabrication technologies. However, the TE-polarized light (the E -field is parallel to the Al wire direction) does not support the excitation of SP modes and thus there is no obvious light conversion process. As a result, the TE-polarized light is strongly suppressed at resonance wavelengths and the transmissions are extremely low. This indicates that such transmission colour filters can simultaneously function as polarizing elements, a highly desirable feature for display applications. Figure 1d shows the simulated time-average magnetic field intensity and electric displacement (arrow) profiles in one MIM stack corresponding to the red spot in Figure 1b . The TM-polarized incident light has a wavelength of 650 nm and the stack period is 360 nm. The magnetic field intensity shows that most of the incident light is coupled into antisymmetric waveguide modes with maximum intensity near the edges of top and bottom Al gratings, which supports our design principle. From the electric displacement, we can see that the efficient coupling of incident light to the SP antisymmetric modes is realized by the strong magnetic response, as in the case of a previous report [22] in which the electric displacement forms a loop and results in strong magnetic fields opposing that of the incident light inside the dielectric layer. 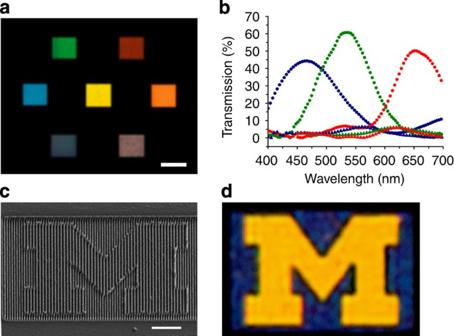Figure 2: Plasmonic colour filters. (a) Optical microscopy images of seven plasmonic colour filters illuminated by white light. Scale bar, 10 μm. (b) Experimentally measured transmission spectra of three fabricated colour filters corresponding to the RGB colours. The circle and triangle correspond to TM and TE illuminations respectively. (c) Scanning electron microscopy image of the pattern 'M' formed by two stack periods. The periods of the navy blue background and the yellow character are 220 and 310 nm, respectively. Scale bar, 3 μm. (d) Optical microscopy image of the pattern illuminated with white light. Figure 2a shows the optical microscopy images of the seven square-shaped plasmonic colour filters illuminated by the white light. The filters are fabricated using focus ion beam milling of a deposited Al/ZnSe/Al stack on an MgF 2 substrate. The colour filters have the stack period changing from 200 to 360 nm, corresponding to the colour from violet to red. All the filters have the same area dimension of about 10 μm × 10 μm. The measured transmission spectra of RGB filters are given in Figure 2b , which agrees well with the simulation results shown in Figure 1c . For TM illumination, stack arrays show the expected filtering behavior with absolute transmission over 50% around the resonant wavelengths, which is several orders of magnitude higher than those of previously reported MIM resonators [13] . This transmission is comparable with the prevailing colourant-based filter used in an LCD panel, but the thickness of the plasmonic device is 1–2 orders of magnitude thinner than that of the colourant one. The relative lower transmission for blue colour is due to the stronger absorption loss of ZnSe in the shorter wavelength range. The full-width at half maximum of the passbands is about 100 nm for all three colours. However, the devices strongly reflect TE-polarized light, as in wire-grid polarizers [27] . Therefore, the transmission of TE-polarized light is suppressed as shown in Figure 2b . This feature indicates that the structure itself can have the roles of colour filter and polarizer simultaneously, which could greatly benefit the LCD by eliminating the need of a separate polarizer layer. In addition, the conductive nature of the Al grating also implies that a separate transparent conductive oxide layer used in LCD module may not be necessary, as was demonstrated in our previous work on metal-wire-based transparent electrodes [28] , [29] . Figure 2: Plasmonic colour filters. ( a ) Optical microscopy images of seven plasmonic colour filters illuminated by white light. Scale bar, 10 μm. ( b ) Experimentally measured transmission spectra of three fabricated colour filters corresponding to the RGB colours. The circle and triangle correspond to TM and TE illuminations respectively. ( c ) Scanning electron microscopy image of the pattern 'M' formed by two stack periods. The periods of the navy blue background and the yellow character are 220 and 310 nm, respectively. Scale bar, 3 μm. ( d ) Optical microscopy image of the pattern illuminated with white light. Full size image Besides the standard square colour filters, one can use different nanoresonator arrays to form arbitrary coloured patterns on a micrometre scale. As a demonstration, a yellow character 'M' in a navy blue background is shown in Figure 2c . The pattern size of the 'M' logo measures only 20 μm × 12 μm and uses two periods: 310 nm for the yellow letter M and 220 nm for the navy blue background. The optical microscopy image of the pattern illuminated with the white light is shown in Figure 2d . A clear-cut yellow 'M' sharply contrasts the navy blue background. It is important to note that the two distinct colours are well preserved even at the sharp corners and boundaries of the two different patterns, which implies that our colour filter scheme can be extended to ultrahigh-resolution colour displays. Next, we address the following question: how many slits are necessary to render the coloured effect? We performed simulation and experiments to investigate the relationship between the slit number and the filtering effect. 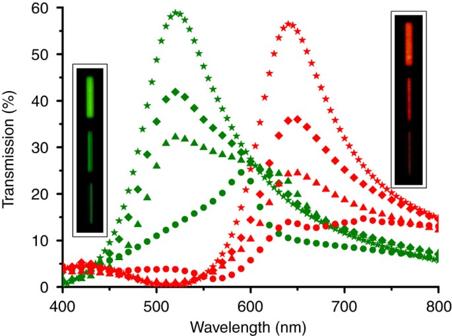Figure 3: Plasmonic colour filters with a few slits. Simulated transmission for the green and red filters with 2, 4, 6 and infinite number of slits. The circle, triangle, diamond and star correspond to the structure with 2, 4, 6 and infinite slits respectively. Inset shows the optical microscopy images for the case of 2, 4 and 6 slits (slit number increases from bottom to top). The inset of Figure 3 shows the microscope images of the samples with 2, 4 and 6 slits (from the bottom to the top) for green and red colour filters. The centre-to-centre distance between the neighbouring slits for green and red filters is 270 and 360 nm, respectively, with slit width about 80 and 100 nm. Amazingly, even the structures with only two slits already exhibit distinct colours. With more slits, the green and red colours become better defined and much brighter, and agree well with the simulation results shown in Figure 3 . This interesting behavior can be explained by the interference of the SP waveguide modes. When the incident light is coupled into the SP modes through the bottom slits, the counterpropagating SP waves inside the insulator layer from different slits would interfere along the waveguide direction, in a manner similar to an earlier work [30] . Transmission will be enhanced for constructive interference at the top slits, and suppressed for destructive interference. Fundamentally, the filtering effect of the stack array with infinite slits can also be ascribed to the multiple interferences of SP waves from each slit. The main difference between structures having a few slits and infinite slits is that the latter can efficiently couple the incident light into SP antisymmetric modes through momentum matching by diffraction, and therefore the efficiency would be much higher. The above analysis and experimental results indicate that very compact structures with just a few slits can still perform the colour-filtering function. Figure 3: Plasmonic colour filters with a few slits. Simulated transmission for the green and red filters with 2, 4, 6 and infinite number of slits. The circle, triangle, diamond and star correspond to the structure with 2, 4, 6 and infinite slits respectively. Inset shows the optical microscopy images for the case of 2, 4 and 6 slits (slit number increases from bottom to top). Full size image Plasmonic nanoresonators for spectral and polarimetric imaging By gradually changing the periods of the plasmonic nanoresonator array, we also design and demonstrate a plasmonic spectroscope for spectral imaging. 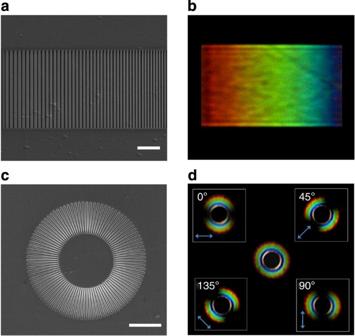Figure 4: Plasmonic spectroscopes for spectral imaging. (a) Scanning electron microscopy (SEM) image of the fabricated 1D plasmonic spectroscope with gradually changing periods from 400 to 200 nm (from left to right). Scale bar, 2 μm. (b) Optical microscopy image of the plasmonic spectroscope illuminated with white light. (c) SEM image of the fabricated 2D spoke structure. Scale bar, 3 μm. (d) Optical microscopy images of the spoken structure illuminated with unpolarized light (centre) and polarized light (four boxes). Figure 4a shows the fabricated device consisting of gradually changing periods from 200 to 400 nm that covers all colours in the visible range. When illuminated with white light, the structure becomes a rainbow stripe, with light emitting from the stack array, as shown in Figure 4b . Plasmonic spectroscopes can disperse the whole visible spectrum in just a few micrometre distance, which is orders of magnitude smaller than the dispersion of the conventional prism-based device. This feature indicates that the colour pixels formed by these structures could provide extremely high spatial resolution for application in multiband spectral imaging systems. In fact, our thin film stack structures can be directly integrated on top of focal plane arrays to implement high-resolution spectral imaging, or to create chip-based ultracompact spectrometers. Figure 4: Plasmonic spectroscopes for spectral imaging. ( a ) Scanning electron microscopy (SEM) image of the fabricated 1D plasmonic spectroscope with gradually changing periods from 400 to 200 nm (from left to right). Scale bar, 2 μm. ( b ) Optical microscopy image of the plasmonic spectroscope illuminated with white light. ( c ) SEM image of the fabricated 2D spoke structure. Scale bar, 3 μm. ( d ) Optical microscopy images of the spoken structure illuminated with unpolarized light (centre) and polarized light (four boxes). Full size image All structures discussed so far only consist of 1D linear slits (that is, a slit in the same direction). Here, we design a 2D microscale spoke structure that has slits in different orientations and a gradual change of slit spacing to further investigate spectral and polarimetric imaging responses. The spoke structure, as depicted in Figure 4c , consists of 96 slits that form a circular ring. Each slit is 3 μm in length and 50 nm in width, and the inner and outer radius of the ring is about 3 and 6 μm. The spacing between neighbouring slits changes from 200 nm from the centre to 400 nm towards the outer edge of the ring, covering all colours in the visible range as the above linear spectroscope. Figure 4d shows the polarimetric response of the spoke with different illuminations. When the spoke is illuminated with unpolarized white light, the transmitted light forms a complete rainbow ring. However, if the illumination is the polarized light and the polarization is rotated, a clear dark region appears along the polarization direction. This is because of the absence of excited SPs in the polarization direction, and thus the transmission is extremely low, which is consistent with the TM coupling discussed earlier. Therefore, this 2D spoke structure, when used with an imaging device, could provide real-time polarimetric information in spectral imaging, or it can be used as a microscale polarization analyser. Human eyes typically have a resolution limit of about 80 μm at 35 mm [31] . Therefore, we can use these plasmonic nanoresonators to build coloured 'super-pixels' that are only several micrometres in a lateral dimension and are much smaller than the resolution limit of the human eyes. At present, this lateral dimension is also 1–2 orders of magnitude smaller than the best high-definition colour filters currently available [32] . Furthermore, these plasmonic devices have a longitudinal thickness that is 1–2 orders of magnitude thinner than that of colourant ones, which is very attractive for the design of ultrathin panel display devices. Besides the small dimensions, the nature of the polarization dependence of plasmonic resonators is also attractive. This feature not only benefits the applications in LCD by eliminating the need of a separate polarizer layer, but can also be used for extracting polarimetric information in spectral imaging. In summary, we proposed and demonstrated plasmonic nanoresonators to disperse light with high efficiency spectrally. By arranging different resonators, arbitrary coloured patterns on a micrometre scale are achievable. These artificial structures provide an opportunity for display and imaging devices with a higher spatial resolution, as well as much smaller device dimensions than those currently available. The design principle can be easily expanded to other wavelength ranges for multispectral imaging. Analytic solution of plasmon dispersion in an MIM structure For TM-polarized waves (the E -field is perpendicular to the Al grating direction), the transverse magnetic plasmon dispersion relation of the MIM structure is given by for the antisymmetric mode, and by for the symmetric mode; k z is defined by the momentum conservation: where ɛ is the complex dielectric constant, subscripts 1 and 2 the insulator and metal layer, and d the thickness of the insulator layer. Here, all materials are assumed to be non-magnetic so that the magnetic permeability is equal to 1. In our case, the Al/ZnSe/Al stack array has a 0.7 duty cycle and therefore the dielectric constant of the insulator layer is calculated following the effective medium theory. The complex dielectric constant of Al is described by fitting the experimentally measured data. The spatial extension of SP waves in the ZnSe layer is calculated to be ∼ 100 nm at visible frequencies. Therefore, we choose a 100 nm-thick ZnSe layer to ensure the efficient coupling of SP modes at the top and bottom edges of the stack. Thereafter, the plasmon dispersions for the antisymmetric and symmetric modes are obtained by solving equations (1) and (2). Device fabrication and measurement A glass substrate was prepared using a cleaning process. A 220 nm magnesium fluoride (MgF 2 ) dielectric layer, 40 nm Al, 100 nm zinc selenide (ZnSe) and another 40 nm Al were deposited sequentially using an electron-beam evaporator with a deposition rate of 0.5 nm s −1 . To prevent the Al from oxidizing, we stored the samples in an oxygen-free glove box before measurement. Patterns were milled with the focus ion beam equipped in a Nova NanoLab DuaLbeam workstation (FEI). Milling was controlled with an AutoFIB program, provided by FEI, capable of controlling all parameters relating to ion and electron beams. The accelerating voltage is 30 kV and current varies from 50 to 100 pA, determined by the feature size. Magnification is from ×6,500 to ×10,000 for patterning. Transmission spectra were measured with an inverted microscope (Nikon TE 300; Nikon), and all optical images were taken with a camera (Nikon D3000; Nikon) mounted on the front port of the microscope. How to cite this article: Xu, T. et al . Plasmonic nanoresonators for high-resolution colour filtering and spectral imaging. Nat. Commun. 1:59 doi: 10.1038/ncomms1058 (2010).